TheArabidopsistranscription factor bZIP11 activates auxin-mediated transcription by recruiting the histone acetylation machinery In higher plants, the hormone auxin orchestrates a diverse array of developmental and environmental responses mainly exerted via transcriptional control. In its absence, auxin-mediated transcription is postulated to be repressed by histone deacetylases, which convert chromatin into a highly packed inactive state. Here we present a converse mechanism where Arabidopsis bZIP11-related basic leucine zipper (bZIP) transcription factors interact via an amino-terminal activation domain with ADA2b adapter proteins to recruit the histone acetylation machinery to specific auxin-responsive genes. Gain, loss-of-function and pharmacological approaches as well as chromatin immunoprecipitation experiments addressing various components of the recruitment and acetylation machinery substantiate the proposed mechanism. Importantly, G-box-related cis -elements, frequently found in auxin-induced promoters, are shown to bind bZIP11-related bZIPs and to function as quantitative modulators of auxin-induced transcription. In conclusion, we describe a regulatory activation mechanism that serves as a rheostat to modulate auxin-mediated responses. Various developmental and growth-related plant processes, such as embryogenesis, root and shoot architecture, organ patterning and vascular development are regulated by the plant hormone auxin [1] , [2] . Moreover, responses to environmental signals such as tropic responses or pathogen defence are associated with this hormone [3] , [4] . To control these various responses, coordinated regulation of auxin-induced genes is required, which is primarily mediated by cis -acting auxin-responsive elements (AuxREs) [5] , [6] , [7] , which are bound by auxin response factors (ARFs) [8] , [9] , [10] . Via protein–protein interaction, ARF-mediated transcription is repressed by AUX/IAA proteins [11] , [12] . These repressors exert their function by interaction with the Groucho/Tup type corepressor TOPLESS that is thought to recruit histone deacetylases (HDACs) to target promoters [13] , [14] leading to transcriptionally inactive, tightly packed chromatin [15] . In response to auxin perception, which is mediated by the F-box protein TIR1, AUX/IAAs are polyubiquitinated by the SCF TIR1 complex and subsequently degraded by the 26S proteasome [16] , [17] . This regulatory mechanism based on derepression enables rapid ARF-mediated gene activation [8] . However, a complementary mechanism leading to activation of auxin-responsive genes via histone acetyltransferases has not been elucidated yet. In Arabidopsis , five HAT genes related to the yeast GCN5 have been described, termed histone acetyltransferase of the GNAT/MYST superfamily (HAG1-5) [15] , [18] , [19] , [20] . GCN5 and the transcription factor (TF) adaptor proteins ADA2b and ADA2a physically interact and are, as shown for their yeast orthologs, components of the Arabidopsis SAGA (Spt/Ada/GCN5/acetyltransferase)-like chromatin remodelling complex [21] . Several data sets support the impact of histone acetylation on auxin signalling. In fact, gcn5 and ada2b mutants, in which SAGA complex formation should be disrupted, exhibit several abnormal auxin-related growth phenotypes [20] , [22] , [23] , [24] . Moreover, GCN5 has been found in a mutant suppressor screen for the corepressor TPL [24] and ADA2b was shown to be required for histone acetylation in response to auxin [25] . Consistently, the ada2b -mutant plants are impaired in translating auxin signals into proper morphogenetic responses [26] . Although indicative of an involvement of histone acetylation and deacetylation in regulating auxin responses, a direct prove disclosing the impact of HAT- and HDAC-mediated chromatin remodelling is still elusive. In order to open up chromatin by acetylation, an adapter is required that binds specifically to a respective auxin-inducible promoter to recruit the histone acetylation machinery. ADA2 proteins are able to interact with DNA-binding TFs, providing a mechanism to recruit HAT-containing SAGA-like complexes [21] . To date, a few direct physical interactions between plant ADA2 homologues and transcriptional activators could be identified. Arabidopsis ADA2b interacts with the AP2 TF CBF1, which promotes expression of several cold-responsive genes [27] , [28] , whereas ADA2 from maize binds the basic leucine zipper (bZIP) factor OPAQUE2 (O2), which is involved in regulating seed storage genes during maize endosperm development [29] , [30] . Auxin-induced transcription has been studied in the context of several rapidly responding groups of genes like SAURs , IAAs and GH3s . Group II GH3 genes encode for enzymes that modify the pool of active auxin by conjugation to amino acids (aa) and hence are crucial regulatory nodes in auxin homeostasis and auxin-related growth responses [31] , [32] . Previous promoter analyses implicate that beside AuxREs, other cis -elements are involved in auxin-mediated transcription. For example, a conserved organization of G-box-related elements (GREs, consensus: BACGTV ) located in close vicinity to AuxREs has been found in soybean and tobacco GH3 promoters [33] , [34] . Moreover, bioinformatic studies reveal an enrichment of modules consisting of GREs and AuxREs in auxin-inducible promoters in Arabidopsis and rice [35] . GREs are typical binding sites for bZIP TFs [36] . Although G-box binding activity has been described with respect to the soybean GH3 promoter, the corresponding TFs have not been assigned yet [37] . However, the tobacco bZIP factors BZI-1 and BZI-2 were found to regulate auxin-mediated NtGH3 transcription [33] , [38] , [39] . In order to identify cis -regulatory elements and trans -binding factors that act as a recruitment platform for the histone acetylation machinery, this work utilizes the Arabidopsis auxin-inducible GH3.3 model promoter to characterize GREs as quantitative modulators of AuxRE-mediated transcription. Screening approaches in protoplasts reveal bZIP11-related TFs that activate GH3.3 expression via GREs. By physical interaction with ADA2b, these bZIPs recruit the SAGA complex via their N-terminal activation domain (AD). Chromatin immunoprecipitation (ChIP) experiments confirm that bZIP binding to the GH3.3 promoter correlates with enhanced GCN5 recruitment, GCN5-specific histone H3K27 acetylation and binding of RNA polymerase II (RNPII). In all, these data provide a mechanistic model describing a bZIP-mediated recruitment of the histone acetylation machinery to activate auxin-induced transcription. Auxin-responsive genes are regulated by histone acetylation To confirm the assumption that auxin-induced transcription is controlled by histone acetylation and deacetylation, we monitored the expression of auxin-responsive marker genes in the absence and presence of the broad-spectrum HDAC inhibitor trichostatin A (TSA) [40] , [41] or the GCN5-specific HAT inhibitor, γ-butyrolactone [42] . To ensure equal exposure of the plant cells to the additives, wild-type (WT) mesophyll protoplasts were prepared and incubated with low concentrations of TSA or γ-butyrolactone, prior to subjection to an additional auxin or mock treatment. As demonstrated in Fig. 1a , TSA induces the transcription of the auxin-responsive marker genes with varying intensities. In particular, the moderately auxin-inducible PIN4 (At2g01420) gene was strongly derepressed by TSA treatment. Moreover, distinct differences in induction were observed after TSA and auxin co-treatment. In contrast to GH3.3 (At2g23170), auxin-induced transcription of IAA3 (At1g04240) and, to a minor extent, of IAA7 (At3g23050) and PIN4 was further enhanced by TSA. 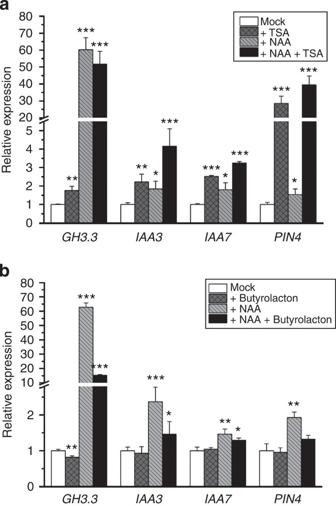Figure 1: Auxin-responsive gene expression is regulated by histone acetylation and deacetylation. Expression of selected auxin-responsive genes was analysed in protoplasts by qRT–PCR in the absence (mock) or presence of auxin (NAA) and (a) the HDAC inhibitor, TSA or (b) the GCN5 inhibitor, γ-butyrolactone. Mock (white), inhibitor (dark grey, chequered), NAA (light grey, fasciated) or NAA and inhibitor (black)-treated samples are presented in differently labelled bars. Given are mean expression levels (±s.e.m.) (n=3) relative to mock-treated samples. Statistical significant differences compared with mock-treated samples were determined by Studentst-test (*P≤0.05; **P≤0.01; ***P≤0.001). Figure 1: Auxin-responsive gene expression is regulated by histone acetylation and deacetylation. Expression of selected auxin-responsive genes was analysed in protoplasts by qRT–PCR in the absence (mock) or presence of auxin (NAA) and ( a ) the HDAC inhibitor, TSA or ( b ) the GCN5 inhibitor, γ-butyrolactone. Mock (white), inhibitor (dark grey, chequered), NAA (light grey, fasciated) or NAA and inhibitor (black)-treated samples are presented in differently labelled bars. Given are mean expression levels (±s.e.m.) ( n =3) relative to mock-treated samples. Statistical significant differences compared with mock-treated samples were determined by Students t -test (* P≤ 0.05; ** P≤ 0.01; *** P≤ 0.001). Full size image To inhibit GCN5-specific histone acetylation, γ-butyrolactone was applied. It has been demonstrated to efficiently target aa within the catalytic active site of the mammalian GCN5 enzyme [42] . As these aa are conserved within the homologous yeast and Arabidopsis proteins ( Supplementary Fig. 1 ) γ-butyrolactone is assumed to be functionally active in plant cells. Application of γ-butyrolactone has no ( IAA3 , IAA7 and PIN4 ) or little effect ( GH3.3 ) on gene induction in the absence of external auxin. However, it significantly reduced auxin-induced transcription of the marker genes when both compounds were applied ( Fig. 1b ). In summary, these pharmacological data clearly underline the involvement of histone acetylation regulating auxin-induced transcription. A 300 bp GH3.3 promoter region mediates auxin responsiveness To define which promoter cis -elements are involved to recruit the histone acetylation machinery, a detailed analysis of the auxin-inducible Arabidopsis GH3.3 promoter has been performed. This promoter was chosen based on its homology to the best characterized auxin-responsive model promoter [34] and due to the finding that its auxin-induced activation strongly depends on histone acetylation ( Fig. 1b ). To perform rapid analyses, the activity of GH3.3 promoter GUS fusions (Pro GH3.3 :GUS) was tested in transiently transformed Arabidopsis protoplasts. Physiological levels of auxin (0.25 μM α-naphthaleneacetic acid, NAA) were sufficient to strongly and reliably induce GH3.3 reporter gene activity. Using a deletion approach ( Fig. 2a ), a nucleotide region ~\n300 bp upstream the ATG start codon was necessary and sufficient to obtain auxin responsiveness comparable with the 1,700 bp full-length GH3.3 promoter. In a complementary approach, neither the −1,700 to −300 bp promoter fragment fused to a minimal promoter nor a mutational derivate lacking all discernible AuxRE cis -elements ( Fig. 2a,b ) conferred any auxin responsiveness to the GUS reporter. These data indicate that the 300 bp sequence proximal to the ATG start codon ( GH3.3 −300 ) is required for the promoters’ auxin responsiveness. 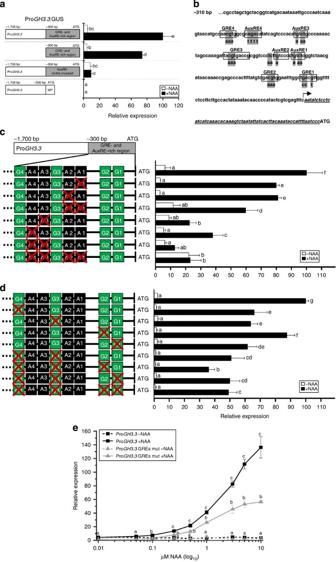Figure 2: Analysis of theGH3.3promoter inArabidopsisprotoplasts. (a) Promoter activity was analysed using reporter:GUS constructs. Results were obtained with the full-length 1,700 bpGH3.3promoter (ProGH3.3−1,700), the 300 bp,cis-element-rich promoter region proximal to the transcriptional start site (TSS) (ProGH3.3−300), a mutational ProGH3.3−1,700derivate that lacks all discernible AuxREcis-elements and the remaining TSS distal promoter fragment (ProGH3.3−300–1,700) fused to a minimal promoter. Promoter activity was analysed in the absence (white) or presence (black bars) of applied NAA. (b) Schematic drawing of theGH3.3−300promotercis-element organization and the mutations applied. The TSS and 5′UTR are indicated by an arrow or shown in italic letters, respectively. (c,d) Expression of the ProGH3.3−1,700:GUS construct and its indicated mutational derivatives was analysed in protoplasts. Results were obtained with mutations in (c) AuxREs (black) and (d) GREs (green). (e) Expression of a ProGH3.3−1,700:GUS reporter (black) and a construct lacking all GREs (grey) was monitored in an auxin concentration-dependent manner. Given are mean expression levels (±s.d.) (n=3) relative to the auxin-inducedGH3.3promoter activity (set to 100%) (a,c,d) or mock-treated samples (e). Significant differences between constructs and treatments were labelled with different letters (one-way analysis of variance followed by Fisherpost hoctest;P<0.05). Figure 2: Analysis of the GH3.3 promoter in Arabidopsis protoplasts. ( a ) Promoter activity was analysed using reporter:GUS constructs. Results were obtained with the full-length 1,700 bp GH3.3 promoter (Pro GH3.3 −1,700 ), the 300 bp, cis -element-rich promoter region proximal to the transcriptional start site (TSS) (Pro GH3.3 −300 ), a mutational Pro GH3.3 −1,700 derivate that lacks all discernible AuxRE cis -elements and the remaining TSS distal promoter fragment (Pro GH3.3 −300–1,700 ) fused to a minimal promoter. Promoter activity was analysed in the absence (white) or presence (black bars) of applied NAA. ( b ) Schematic drawing of the GH3.3 −300 promoter cis -element organization and the mutations applied. The TSS and 5′UTR are indicated by an arrow or shown in italic letters, respectively. ( c , d ) Expression of the Pro GH3.3 −1,700 :GUS construct and its indicated mutational derivatives was analysed in protoplasts. Results were obtained with mutations in ( c ) AuxREs (black) and ( d ) GREs (green). ( e ) Expression of a Pro GH3.3 −1,700 :GUS reporter (black) and a construct lacking all GREs (grey) was monitored in an auxin concentration-dependent manner. Given are mean expression levels (±s.d.) ( n =3) relative to the auxin-induced GH3.3 promoter activity (set to 100%) ( a , c , d ) or mock-treated samples ( e ). Significant differences between constructs and treatments were labelled with different letters (one-way analysis of variance followed by Fisher post hoc test; P <0.05). Full size image Non-redundant AuxREs regulate Pro GH3.3 auxin responsiveness The Arabidopsis GH3.3 −300 promoter region harbours multiple redundant cis -elements. In particular, four AuxREs were identified that display a TGTCTC (AuxRE1) or TGTCTG (AuxRE3, AuxRE4) consensus [5] and a related TGTCCC motif (AuxRE2) ( Fig. 2b ). The AuxRE1 and AuxRE2 constitute a module organized as a tandem direct repeat. To reveal the functional impact of the AuxRE elements, an analysis of the GH3.3 −1,700 promoter was performed in protoplasts making use of the mutations shown in Fig. 2b . As demonstrated in Fig. 2c , mutations in either AuxRE1 or AuxRE2 caused a reduction of the Pro GH3.3 auxin inducibility by 20%, whereas both mutations resulted in an additive effect. In contrast, single mutations in AuxRE3 or AuxRE4 reduced auxin responsiveness to 20–40 %. Combined mutation of these or all AuxREs led to a complete loss of auxin-induced GH3.3 promoter activity. Interestingly, the AuxRE1–4 mutation led to a slightly increased basal GUS level, indicating that AuxREs are occupied by repressive ARF/IAA complexes. In summary, although all AuxREs participate in auxin responsiveness, AuxRE3 and AuxRE4 are the most crucial cis -elements in the GH3.3 promoter. GREs quantitatively regulate auxin-induced transcription Based on the hypothesis that further cis -elements are involved in recruiting the histone acetylation machinery, we focused our studies on GREs, which are found to be enriched in auxin-induced promoters [35] and have been implicated in auxin-induced transcription [33] , [34] . Two GREs were identified in the GH3.3 promoter, named GRE2 (GACGTG) and GRE4 (AACGTG), whereas GRE1 and GRE3 were found to overlap with TGACG motifs. Both types of cis -elements are recognized by G-box binding factors, whereas the latter is known to be the typical binding site for group D bZIPs [43] . A detailed mutational analysis based on the Pro GH3.3 −1,700 sequence revealed that single mutations in GREs ( Fig. 2d ) reduced the activity of the GH3.3 reporter construct by 20– 40%. Generally, an increasing number of mutated GREs reduced the level of auxin-induced GH3.3 expression in a non-additive way. Importantly, mutations in multiple GREs did not completely impair responsiveness of the GH3.3 promoter to auxin. A threshold induction of ~\n50% remained when all GREs were mutated. These data demonstrate that despite their qualitative function, the AuxREs are not sufficient to provide full auxin inducibility on their own. To further analyse the biological impact of GREs, we conducted an auxin dose-response study comparing the genuine and the GRE mutated Pro GH3.3 :GUS construct ( Fig. 2e ). Interestingly, GREs have a more pronounced input on auxin-mediated transcription at higher auxin concentrations, highlighting their role as quantitative cis -elements. In order to address a putative functional link between the most relevant AuxRE3/4 and a particular GRE, we reduced the complexity of the GH3.3 promoter by mutating the tandem AuxRE1/2 motif ( Supplementary Fig. 2a ). An additional single mutation of any GRE led to a similar reduction in auxin responsiveness, indicating that the GREs are functionally equivalent and that all GREs cooperate with AuxRE3 and AuxRE4 in auxin-mediated transcription of the GH3.3 promoter. Due to their quantitative impact on auxin-induced transcription and their functional interplay with AuxREs, GREs are well-suited candidates to act as docking platforms for proteins recruiting the acetylation machinery. Specific C/S bZIPs enhance auxin-induced GH3.3 transcription Previous work in tobacco has proposed bZIP TFs to regulate NtGH3 transcription via GREs [33] . We therefore studied the activation properties of nine homologous Arabidopsis group C and S1 bZIP factors ( Fig. 3a ). Group S1 bZIP2 (At2g18160), -11 (At4g34590), -44 (At1g75390), -53 (At3g62420) and the group C factor bZIP63 (At5g28770) specifically enhanced auxin-mediated Pro GH3.3 −1,700 :GUS expression, whereas other bZIPs, such as bZIP1 (At5g49450), bZIP9 (At5g24800) or bZIP10 (At4g02640), had no impact. Notably, bZIP-enhanced GH3.3 reporter activity was not only observed when auxin was applied but also seen in the noninduced control samples. 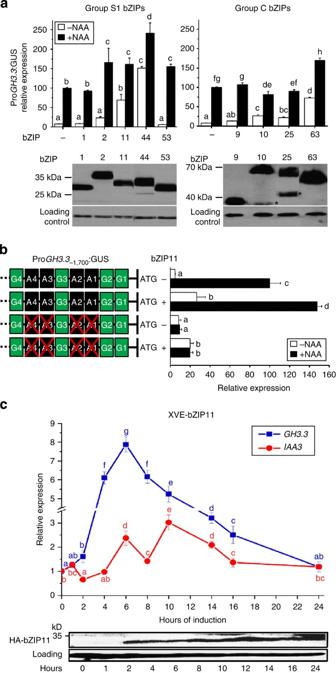Figure 3: Particular bZIP TFs of the C/S1 network regulateGH3.3 expression. (a) Activation of the ProGH3.3−1,700:GUS reporter was measured in protoplasts in the absence (white) or presence (black bars) of applied NAA and/or after coexpression of bZIPs. Expression of the HA-tagged bZIP effectors was confirmed by immunodetection. Asterisks mark degradation products. (b) Activation potential of bZIP11 on the genuine ProGH3.3−1,700:GUS reporter or a derivative harbouring mutations in all AuxREs was analysed in protoplasts. GRE or AuxREcis-elements are presented as green or black boxes, respectively. Mutations are indicated by X. Given are mean expression levels (±s.d.) (n=3) relative to the induction of theGH3.3promoter (100%). (c) Transcription ofGH3.3(blue square) and IAA3(red circle) was studied by qRT−PCR in transgenic XVE-bZIP11 plants that express HA-bZIP11 in an Est-dependent manner. Presented are the mean fold expression levels (±s.e.m.) (n=3) compared with uninduced plants obtained after the induction time points indicated. Expression of HA-tagged bZIP11 proteins was analysed by immunodetection. Significant differences between treatments are designated by different letters (one-way analysis of variance with Fisherpost hoctest;P<0.05). Figure 3: Particular bZIP TFs of the C/S1 network regulate GH3.3 expression. ( a ) Activation of the Pro GH3.3 −1,700 :GUS reporter was measured in protoplasts in the absence (white) or presence (black bars) of applied NAA and/or after coexpression of bZIPs. Expression of the HA-tagged bZIP effectors was confirmed by immunodetection. Asterisks mark degradation products. ( b ) Activation potential of bZIP11 on the genuine Pro GH3.3 −1,700 :GUS reporter or a derivative harbouring mutations in all AuxREs was analysed in protoplasts. GRE or AuxRE cis -elements are presented as green or black boxes, respectively. Mutations are indicated by X. Given are mean expression levels (±s.d.) ( n =3) relative to the induction of the GH3.3 promoter (100%). ( c ) Transcription of GH3.3 (blue square) and I AA3 (red circle) was studied by qRT−PCR in transgenic XVE-bZIP11 plants that express HA-bZIP11 in an Est-dependent manner. Presented are the mean fold expression levels (±s.e.m.) ( n =3) compared with uninduced plants obtained after the induction time points indicated. Expression of HA-tagged bZIP11 proteins was analysed by immunodetection. Significant differences between treatments are designated by different letters (one-way analysis of variance with Fisher post hoc test; P <0.05). Full size image In order to analyse the interplay of the GRE/bZIP11 module and the AuxREs, we analysed GH3.3 promoter derivatives, showing mutations in specific ( Supplementary Fig. 2b ) or all four AuxREs ( Fig. 3b ). Without auxin treatment, bZIP11 could activate the Pro GH3.3 −1,700 :GUS reporters independently of the presence of these AuxREs to a comparable level. However, auxin-induced reporter activity, which was dependent on AuxREs, could be further enhanced by bZIP11 expression. This held particularly true for the AuxRE3-mutant construct that was not significantly auxin inducible, whereas bZIP11 coexpression restored auxin inducibility ( Supplementary Fig. 2b ). Altogether, these findings support the quantitative input of the GRE/bZIP module on auxin-mediated transcription. In summary, several, presumably redundant, group S1 bZIP factors quantitatively modulate GH3.3 promoter activity in protoplasts. bZIP11 controls auxin-induced gene expression in planta As bZIP11 and -44 showed the strongest activation potential on the GH3.3 promoter in protoplasts, we focused on these TFs applying stably transformed gain-of-function plants. Because constitutive ectopic expression of bZIP11-related bZIPs strongly interferes with plant growth [44] , [45] , we expressed the bZIPs as HA-tagged versions using a β-estradiol (Est)-inducible expression system (XVE) [46] . Quantitative real-time PCR (qRT–PCR) analysis revealed that GH3.3 induction correlated with an early increase of the bZIP11 regulator, which becomes detectable by immunoblot after 2 h of Est treatment ( Fig. 3c ). However, GH3.3 transcript accumulation that peaked around 6 h post induction was transient, presumably due to bZIP11-mediated coactivation of IAA repressors ( Fig. 3c , Supplementary Fig. 3b ). Although differences in kinetics have been observed, other tested auxin-induced genes (for example, GH3.5 (At4g27260) and IAA29 (At4g32280)) ( Supplementary Fig. 3a–d ) follow a similar induction pattern, indicating a broader impact of bZIP11 on auxin-induced gene expression. However, it has to be pointed out that only specific auxin-induced genes are regulated. Similar results were obtained with Est-inducible expression of bZIP44, indicating a related function ( Supplementary Fig. 3e ). Importantly, control experiments demonstrate that the application of Est had no effect on target gene transcription ( Supplementary Fig. 3f ). bZIP11 interacts with the histone acetylation machinery Based on the observation that the induction capacity of bZIP11 on GH3.3 and IAA3 correlates with the genes’ dependency on histone acetylation ( Figs 1b and 3c ), we tested whether bZIP11-related bZIPs are able to recruit the histone acetylation machinery to open up packed chromatin. Using a protoplast two hybrid approach (P2H) [47] , a significant interaction between ADA2b (At4g16420) and the closely related group S1 members bZIP2, -11 and -44 and group C bZIP10 and -25 could be identified ( Fig. 4a ). Using the ADA2b homologue ADA2a (At3g07740) as bait in this system, a considerably weaker interaction with bZIP2, -11 and -44 and hardly any with the group C bZIPs could be determined ( Supplementary Fig. 4a ). To validate the data obtained by P2H, co-immunoprecipitation (Co-IP) studies were performed by expressing HA-tagged bZIPs and MYC-tagged ADA2b in Arabidopsis mesophyll protoplasts. Applying an α-HA antibody, ADA2b-MYC protein was efficiently recovered from samples expressing group S1 HA-bZIP2, -11, -44 and HA-bZIP10 or -25 ( Supplementary Fig. 4b ). Hardly any interaction could be determined for bZIP63, which is in line with the results obtained by P2H. In conclusion, these results support the hypothesis that the transactivation properties of these bZIPs are at least in part dependent on the recruitment of the SAGA complex, which is mediated in particular by interaction with the ADA2b adapter protein. 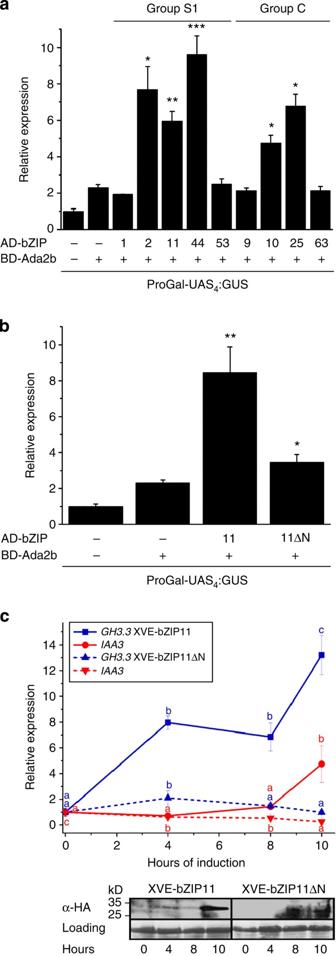Figure 4: Specific bZIP TFs are able to bind the HAT complex adapter protein ADA2bin vivo. (a) Binding of bZIPs to ADA2b was analysed in protoplast two hybrid assays. Presented are mean values (±s.d.) (n=3) relative to the ProGal4-UAS:GUS background. (b) The N terminus of bZIP11 is crucial for ADA2b binding. ADA2b binding capacity of full-length and N-terminally truncated bZIP11 was analysed in P2H assays. Expression of full-length and N-terminally truncated HA-tagged proteins was analysed by immunodetection (see inset). Results are given as mean relative expression values (±s.d.) (n=3). Significant differences between BD-ADA2b driven expression and specific BD/AD combinations were determined by Studentst-test (*P≤0.05; **P≤0.01; ***P≤0.001). (c) Transactivation properties of full-length and N-terminally truncated bZIP11 were studied in transgenic XVE plants. Expression ofGH3.3(blue square) orIAA3(red circle) was analysed by qRT–PCR. Presented are the mean fold expression levels (±s.e.m.) (n=3) compared with uninduced plants obtained after the induction time points indicated. Expression of full-length and truncated HA-tagged bZIP11 protein was analysed by immunodetection. Significant differences between treatments are designated by different letters (one-way analysis of variance with Fisherpost hoctest;P<0.05). Figure 4: Specific bZIP TFs are able to bind the HAT complex adapter protein ADA2b in vivo . ( a ) Binding of bZIPs to ADA2b was analysed in protoplast two hybrid assays. Presented are mean values (±s.d.) ( n =3) relative to the ProGal4-UAS:GUS background. ( b ) The N terminus of bZIP11 is crucial for ADA2b binding. ADA2b binding capacity of full-length and N-terminally truncated bZIP11 was analysed in P2H assays. Expression of full-length and N-terminally truncated HA-tagged proteins was analysed by immunodetection (see inset). Results are given as mean relative expression values (±s.d.) ( n =3). Significant differences between BD-ADA2b driven expression and specific BD/AD combinations were determined by Students t -test (* P≤ 0.05; ** P≤ 0.01; *** P≤ 0.001). ( c ) Transactivation properties of full-length and N-terminally truncated bZIP11 were studied in transgenic XVE plants. Expression of GH3.3 (blue square) or IAA3 (red circle) was analysed by qRT–PCR. Presented are the mean fold expression levels (±s.e.m.) ( n =3) compared with uninduced plants obtained after the induction time points indicated. Expression of full-length and truncated HA-tagged bZIP11 protein was analysed by immunodetection. Significant differences between treatments are designated by different letters (one-way analysis of variance with Fisher post hoc test; P <0.05). Full size image The N-terminus of bZIP11 is crucial for ADA2b interaction The N terminus of bZIP11 or bZIP44 is characterized by several polar and acidic aa ( Supplementary Fig. 4c ). As these residues frequently serve as interaction surfaces [48] and due to their absence in the closely related, non-interacting proteins bZIP53 and bZIP1, we hypothesized that the bZIPs’ N-terminal regions (26 aa in bZIP11 or 40 aa in bZIP44) may function as ADA2 interaction domains. To test this assumption, N-terminally truncated bZIP11 and -44 effector constructs were generated and binding of the full-length and truncated proteins to ADA2b was analysed in P2H studies. A deletion of the N-terminal domain of bZIP11 ( Fig. 4b ) and -44 ( Supplementary Fig. 4d ) strongly compromised their capacity to bind ADA2b. To examine the transactivation properties of truncated bZIP11, target gene expression was analysed in XVE-HA-bZIP11 and XVE-HA-bZIP11ΔN plants ( Fig. 4c ). Although immunodetection confirmed equal expression of bZIP11 and truncated bZIP11ΔN, GH3.3 was significantly less induced and IAA3 even repressed by the truncated TF. Hence, the N-terminal interaction surface is crucial for bZIP11 function as a transcriptional activator. Similar results were obtained for bZIP44ΔN in transiently transformed protoplasts ( Supplementary Fig. 4e ). In summary, these results suggest that the N terminus of bZIP11-related TFs acts as an AD by recruiting the histone acetylation machinery via the ADA2b adapter protein. The bZIP/HAT complex regulates auxin-mediated transcription In order to confirm the pharmacologically based results that expression of auxin-regulated genes is dependent on proper HAT activity and that bZIP11-related TFs are involved in HAT recruitment several reverse genetic approaches were pursued. Expecting partial redundancy between bZIP11-related bZIPs, an Est-inducible artificial microRNA (amiRNA) approach in transgenic plants was applied, which significantly reduced the transcript quantity of all three bZIPs (bZIP2/-11/-44) and attenuated the auxin-induced expression of their putative target genes ( Fig. 5a ). Furthermore, Arabidopsis ada2b and gcn5 (At3g54610) mutants were used to disrupt the histone acetylation machinery. QRT–PCR analyses revealed that both mutants concurrently show a substantial reduction in transcript abundance of IAA3 and enhanced expression of GH3.3 ( Fig. 5b,c ). As IAA3 is a potent negative regulator of GH3.3 ( Supplementary Fig. 5 ), it can be assumed that GH3.3 transcription is constitutively derepressed and hence independent on HAT activity in these mutants. In accordance with the hypothesis that ADA2a and ADA2b are thought to have distinct biological functions [49] , expression of GH3.3 and IAA3 are not significantly changed in ada2a -mutant plants ( Fig. 5d ). In conclusion, various genetic approaches disrupting the bZIP11-ADA2b-GCN5 interaction compromise auxin-regulated gene expression. 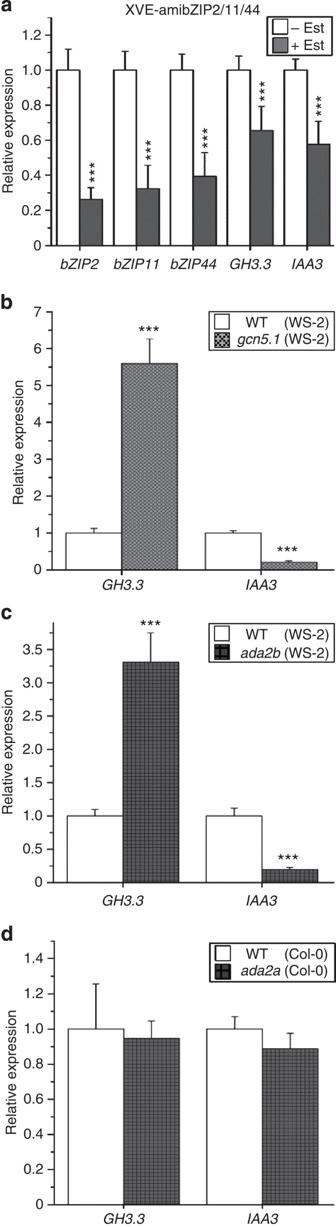Figure 5: Auxin-responsive genes are regulated by bZIP11-related TFs and components of theArabidopsisSAGA-like acetylation complex. (a) Auxin-inducedGH3.3andIAA3transcription was analysed by qRT–PCR in estradiol-inducible bZIP amiRNA knockdown plants (XVE-amiRNA2/11/44, line 2). Mock (white) or Est (grey)-treated samples are visualized by differently coloured bars. (b,d) Expression of the auxin-responsiveGH3.3andIAA3genes was quantified by qRT–PCR in the (b) HAT mutantgcn5-1(light grey, chequered) or mutants in the adaptors (c) ADA2b (dark grey, chequered) or (d) ADA2a (dark grey, chequered), respectively. Given are the mean expression levels (±s.e.m.) (n=3) relative to the corresponding WT or uninduced XVE lines (white bars). Significant differences between WT and mutants or uninduced and induced XVE plants are defined by Studentst-test (*P≤0.05; **P≤0.01; ***P≤0.001). Figure 5: Auxin-responsive genes are regulated by bZIP11-related TFs and components of the Arabidopsis SAGA-like acetylation complex. ( a ) Auxin-induced GH3.3 and IAA3 transcription was analysed by qRT–PCR in estradiol-inducible bZIP amiRNA knockdown plants (XVE-amiRNA2/11/44, line 2). Mock (white) or Est (grey)-treated samples are visualized by differently coloured bars. ( b , d ) Expression of the auxin-responsive GH3.3 and IAA3 genes was quantified by qRT–PCR in the ( b ) HAT mutant gcn5-1 (light grey, chequered) or mutants in the adaptors ( c ) ADA2b (dark grey, chequered) or ( d ) ADA2a (dark grey, chequered), respectively. Given are the mean expression levels (±s.e.m.) ( n =3) relative to the corresponding WT or uninduced XVE lines (white bars). Significant differences between WT and mutants or uninduced and induced XVE plants are defined by Students t -test (* P≤ 0.05; ** P≤ 0.01; *** P≤ 0.001). Full size image bZIP11 activates auxin-responsive genes by HAT recruitment Transcriptionally active chromatin is associated with acetylation of specific lysine residues in the N-terminal tail of histone 3, namely K9, K14 and K27. This is thought to enhance the accessibility of the DNA for trans -acting co-activators, thereby facilitating transcription [50] , [51] . As bZIP11 and -44 recruit the SAGA complex in a sequence-specific manner, we posed the question if enhanced bZIP binding to the GH3.3 promoter correlates with its enhanced GCN5-specific histone acetylation and RNPII recruitment. To address this issue, ChIP analyses of uninduced and Est-induced XVE-HA-bZIP11 and XVE-HA-bZIP44 plants were performed applying specific antibodies. These were raised against HA-tagged bZIP fusion proteins, GCN5-specific lysine 27 acetylation of histone 3 and the activated, C-terminally phosphorylated RNPII. As bZIP11-related TFs preferably bind to GREs and envisaged bZIP-mediated histone acetylation and RNPII binding should also occur in this region, we quantified for each individual ChIP assay the immunoprecipitated GRE-rich GH3.3 promoter region by qRT–PCR ( Fig. 6a ). PCR products derived from the non-bZIP binding GH3.3 coding region or ACTIN7 (At5g09810) promoter were used as negative controls. By this means, we could demonstrate that an Est-induced expression obtained after 6 h ( Fig. 3c ) of either HA-bZIP11 or HA-bZIP44 results in an enhanced binding of the HA-tagged bZIP ( Fig. 6b ), a strongly elevated GCN5-specific H3K27 acetylation ( Fig. 6c ) and a significantly increased assembly rate of the activated RNPII complex on the GH3.3 promoter ( Fig. 6d ). Using the same experimental setup, ChIP assays were performed applying a GCN5-specific antiserum [18] . The obtained data finally demonstrate that bZIP11-related expression directly correlates with GCN5 recruitment to the GH3.3 promoter ( Supplementary Fig. 6 ). In conclusion, these in vivo data clearly propose that bZIP11 and bZIP44 activate transcription of this auxin-responsive gene by chromatin remodelling. 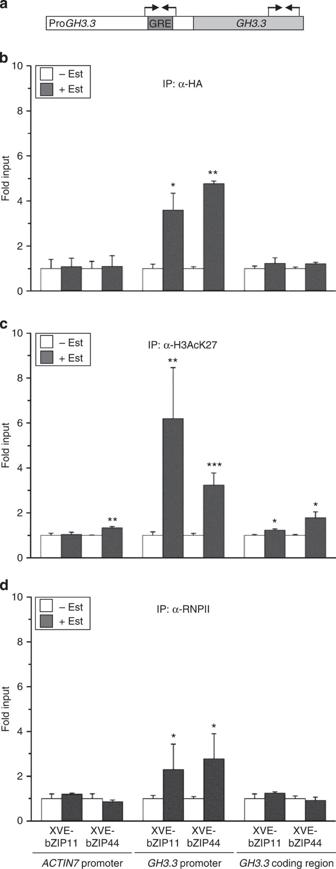Figure 6: bZIP binding to theGH3.3promoter correlates with enhanced GCN5-specific histone acetylation and RNPII recruitment. ChIP assays were performed (a) on theGH3.3promoter using high-affinity ChIP grade antibodies raised against (b) HA-tagged bZIP11 or -44, (c) GCN5-specific histone 3 lysine 27 acetylation (H3AcK27) and (d) the active RNA polymerase II (serine 5 phosphorylated RPB1 subunit). The amount of the immunoprecipitated GRE-richGH3.3promoter, theGH3.3coding region and the GRE-lessACTIN7promoter was quantified by qRT–PCR for each antibody used. Given is the mean abundance of precipitated DNA fragments (±s.e.m.) (n=2–3) in induced (6 h, 10 μM Est) (grey bars) XVE-bZIP11 or XVE-bZIP44 plants relative to uninduced plants (white bars). Significant differences between uninduced and induced samples are defined by Studentst-test (*P≤0.05; **P≤0.01; ***P≤0.001). Figure 6: bZIP binding to the GH3.3 promoter correlates with enhanced GCN5-specific histone acetylation and RNPII recruitment. ChIP assays were performed ( a ) on the GH3.3 promoter using high-affinity ChIP grade antibodies raised against ( b ) HA-tagged bZIP11 or -44, ( c ) GCN5-specific histone 3 lysine 27 acetylation (H3AcK27) and ( d ) the active RNA polymerase II (serine 5 phosphorylated RPB1 subunit). The amount of the immunoprecipitated GRE-rich GH3.3 promoter, the GH3.3 coding region and the GRE-less ACTIN7 promoter was quantified by qRT–PCR for each antibody used. Given is the mean abundance of precipitated DNA fragments (±s.e.m.) ( n= 2–3) in induced (6 h, 10 μM Est) (grey bars) XVE-bZIP11 or XVE-bZIP44 plants relative to uninduced plants (white bars). Significant differences between uninduced and induced samples are defined by Students t -test (* P≤ 0.05; ** P≤ 0.01; *** P≤ 0.001). Full size image A general characteristic of promoters is their complex composition of regulatory cis -elements, which provides means to integrate various signalling inputs to establish specific expression patterns. Although AuxREs are well-defined auxin-dependent ‘on–off switches’, further cis -elements are required to quantitatively modulate expression according to environmental or developmental cues. As summarized in Fig. 7 , this work identifies the GRE cis -element and its cognate bZIP TFs to function as a ‘rheostat’ modulating AuxRE-mediated transcription and reveals the gene activation mechanism, namely by opening up tightly packed chromatin via bZIP-mediated recruitment of the SAGA-like histone acetylation machinery. 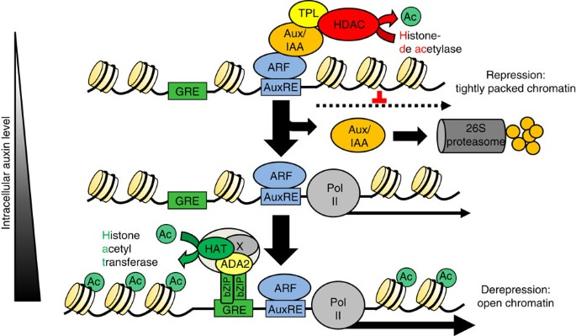Figure 7: Proposed model of the function of bZIP TFs in auxin-mediated transcription. Under auxin-deficient conditions, expression of auxin-responsive genes is repressed by Aux/IAA proteins, which recruit via TOPLESS (TPL) specific HDACs to their target promoters. As soon as auxin concentrations increase Aux/IAA repressor proteins are polyubiquitinated via the SCFTIR1complex and degraded by the 26S proteasome. Aux/IAA degradation derepresses ARF-TF activity enabling target gene expression. In particular, group S1 bZIP TFs are able to boost auxin-mediated transcription by ADA2b-mediated recruitment of SAGA-like histone acetyltransferase complexes. Figure 7: Proposed model of the function of bZIP TFs in auxin-mediated transcription. Under auxin-deficient conditions, expression of auxin-responsive genes is repressed by Aux/IAA proteins, which recruit via TOPLESS (TPL) specific HDACs to their target promoters. As soon as auxin concentrations increase Aux/IAA repressor proteins are polyubiquitinated via the SCF TIR1 complex and degraded by the 26S proteasome. Aux/IAA degradation derepresses ARF-TF activity enabling target gene expression. In particular, group S1 bZIP TFs are able to boost auxin-mediated transcription by ADA2b-mediated recruitment of SAGA-like histone acetyltransferase complexes. Full size image Several biased and unbiased bioinformatic approaches have revealed that GREs, which are preferred binding sites for plant bZIP TFs, are significantly enriched in auxin-responsive promoters and are preferentially located in close vicinity to AuxREs [35] , [52] , [53] . Although GREs by themselves are not sufficient to mediate auxin responsiveness, this work demonstrates that GREs cooperate with AuxREs and that they significantly enhance auxin-mediated transcription in an auxin concentration-dependent manner. Hence, GREs act as quantitative coupling elements of AuxRE-mediated transcription. Redundancy of GREs appears to be an important characteristic as multiple copies are found within the GH3.3 promoter and in those of other auxin-induced genes [35] . Although auxin-induced transcription is affected more strongly when several GREs are mutated, GREs function in a non-additive fashion. In conclusion, these results support the proposed regulatory mechanism based on histone modification. In line with our previous findings on tobacco bZIP factors [33] , [39] , we could demonstrate that the homologous Arabidopsis group S1 TFs bZIP2, -11 and -44 boost GH3.3 transcription both after external auxin-induction and under low endogenous auxin levels, indicating that bZIPs sensitize auxin responsiveness. As not all tested bZIPs activate the GH3.3 promoter, their function is clearly specific. Importantly, studies on several well-known auxin-induced gene families revealed a selective impact of bZIP11-related TFs on a particular subset of these genes. As exemplified in the data set, it remains to be studied why specifically two out of four tested GH3 genes are controlled by bZIP11. The observation that GREs are frequently found in auxin-induced promoters suggests that additional TFs might use the GRE gateway to integrate various signalling inputs into auxin-induced transcription. The bZIP factors studied here belong to the C/S1 network of bZIP TFs that have been demonstrated to form specific heterodimers and to be involved in reprogramming of metabolism in response to low energy stress [45] , [54] , [55] , [56] . Hence, it is tempting to speculate, that the described regulatory mechanism is used to adjust auxin-mediated responses to the energy status of the cell. However, further studies are needed to elucidate the functional impact of these transcriptional regulators. Making use of pharmacological and genetic approaches, we demonstrate that chromatin remodelling by histone acetylation and deacetylation is a crucial mechanism in auxin-regulated transcription. Inhibition of HDACs by TSA derepresses transcription of selected auxin-induced marker genes. However, significant quantitative differences have been observed, underlining the impact of promoter-specific properties. These could be promoter-specific regulation by distinct HDACs that exhibit individual sensitivities to TSA or that TSA-mediated HDAC inactivation is insufficient to completely derepress certain target promoters. In contrast to TSA, inhibition of acetylation by a GCN5-specific HAT inhibitor represses auxin-induced transcription, which is in line with the model that their auxin-mediated expression is facilitated by a HDAC counteracting system. As members of the GH3 , IAA and PIN gene families are regulated in a similar manner, we assume a more general impact of histone acetylation on auxin-mediated gene expression. In fact, recently published results highlight the relevance of ADA2b and GCN5 on auxin-regulated transcription [24] , [25] . GRE/bZIP-mediated recruitment of the SAGA acetylation machinery provides an efficient mechanism to explain the quantitative impact of the GRE/bZIP module on auxin-induced transcription. Using in vivo P2H and Co-IP studies, bZIP11-related bZIPs were in fact found to directly interact with ADA2b, an important TF adapter component of the SAGA complex. Comparing several bZIP factors in interaction assays, we could demonstrate that the ADA2b recruitment is not restricted to bZIP11-related group S1 bZIPs, but is conserved among some group C members as well. In this respect, the Arabidopsis group C members bZIP10 and -25 also interact with the ADA2b protein, as it has been shown for the closely homologous maize bZIP O2 (refs 29 , 30 ). Interestingly, recent publications implicate seed-specific gene regulation with histone acetylation and show that O2 and bZIP10 or bZIP25 (At3g54620) exert related functions in regulation of seed storage protein genes in maize and Arabidopsis [30] , [44] . Hence, these data suggest that bZIPs are not only involved in recruiting the acetylation machinery during auxin-induced transcription. As GREs frequently act as quantitative cis -elements in a wide array of stimulus-induced gene expressions [36] , [44] , [54] , [55] , it is tempting to speculate that GRE-mediated recruitment of SAGA complexes has a broader impact on gene regulation. Interestingly, the recruitment properties of the bZIPs for specific adapter proteins differ. For example, bZIP11-related TFs recruit both ADA2b and ADA2a, although with significant lower affinity for the latter. In contrast, adapter binding of bZIP10/-25 appears to be only specific to ADA2b. Accordingly, expression of auxin-induced genes is not affected in ada2a mutants but strongly impaired in ada2b. Moreover, auxin-related phenotypic alterations are only pronounced in ada2b mutants, which cannot be rescued by ADA2a expression [20] , [49] . Further studies are needed to disclose whether by combinatorial means specific SAGA-like protein complexes are formed that address distinct sets of targets. In contrast to bZIP53 and bZIP1 that do not interact with ADA2b, bZIP11 and bZIP44 share a similar N-terminal domain. In fact, N-terminally truncated derivatives of bZIP11 and -44 exhibit a significantly reduced capacity to bind ADA2b and to promote transcription of their auxin-responsive target genes. Hence, providing a protein–protein interaction platform these N-terminal regions function as transcriptional ADs. As amino-acid alignments of the N-terminal bZIP domains did not reveal strictly conserved motives, the interaction platform is probably characterized by biochemical features, such as polar, acidic residues that are frequently found in eukaryotic ADs [48] . As overexpression of TFs might lead to artificial binding to promoters or interactions with co-regulators, complementary loss-of-function approaches are needed to validate the given hypothesis. For this reason, we employed mutants or inducible amiRNA lines that interfere with components of the HAT complex or HAT recruitment machinery, respectively. In line with the proposed model, these approaches led to a strong impairment of auxin-induced expression. This is particularly true for approaches targeting bZIP2/-11/-44 , ADA2b or GCN5 expression. Comparing auxin-induced expression of GH3.3 and IAA3 in ada2b and gcn5 -mutant lines revealed the same pattern, supporting a model that both proteins functionally cooperate in the SAGA complex. Unexpectedly, GH3.3 expression is strongly enhanced in the gcn5 and ada2b mutants, whereas expression of IAA3 is significantly reduced. In fact GH3.3 expression seems to be strongly repressed by IAA3 ( Supplementary Fig. 5 ). Consequently, the low level of IAA3 expression in the gcn5 and ada2b mutants results indirectly in constant derepression of GH3.3 , which is no longer dependent on the counteracting GCN5/ADA2b histone acetylation machinery. Due to this observation, the significance of GCN5 on GH3.3 expression is hard to address by this mutant analysis. However, the short-term pharmacological approaches that are well suited to analyse more direct effects on gene regulation clearly demonstrate that auxin-induced GH3.3 expression is dependent on proper GCN5 activity. The mechanistic model based on pharmacological, biochemical and reverse genetic data was further supported by in vivo experiments on transcriptional regulation. ChIP analyses confirmed that Est-induced bZIP expression leads to an enhanced binding of the HA-tagged bZIP11 and bZIP44 to the GH3.3 promoter sequence, which harbours several GRE binding sites. This binding coincides with enhanced GCN5 recruitment, GCN5-specific histone 3, lysine 27 acetylation and assembly of RNPII, which consequently results in enhanced transcription of GH3.3 . As summarized in Fig. 7 , this work complements the current model of auxin-mediated transcription. Although AuxREs function as sufficient ‘on–off’ switches, we provide a detailed mechanistic description of a GRE-coupling element, which quantitatively enhances auxin-induced transcription by bZIP-mediated SAGA recruitment to accomplish chromatin remodelling. However, future studies are needed to disclose how individual TF adapters and SAGA-like complexes are employed to gain specificity in auxin-mediated transcriptional regulation. Derepression of transcription by hormone-driven degradation of repressor/HDAC complexes is a characteristic feature of several hormone signalling pathways. As our work constitutes a basic paradigm of a HDAC counteracting mechanism, it will be of great interest to analyse if these hormone responses can also be actively and quantitatively modulated by adapter-mediated HAT recruitment. Plant material and culture Ada2a-3 , ada2b-1 and gcn5-1 mutant plants have been characterized in detail [20] , [49] and were cultivated with the respective Arabidopsis thaliana ecotypes Columbia (Col-0) or Wassilewskija (WS-2) on soil under long-day conditions (16 h light /8 h dark) at 23 °C and a relative humidity of 60%. The genotype of all mutant plants was confirmed by PCR using gene- and T-DNA-specific primers ( Supplementary Table 1 ). Transgenic lines were generated using the ‘floral dip transformation’ technique applying the Agrobacterium tumefaciens strain GV3101 [57] . For expression analyses of transgenic XVE lines, surface-sterilized and stratified seeds were cultivated on ¼ MS [58] agar plates without sugars under long-day conditions. Prior to expression analysis by qRT–PCR 2-week old Est-inducible plants were treated with 7–10 μM Est (17-ß-estradiol, E2758, Sigma-Aldrich Chemie, Munich, Germany) in PBS or an appropriate mock solution for time points indicated. For expression analysis of XVE-amiRNA-bZIP2/11/44 lines, the plants were preinduced with 10 μM Est for 20 h to ensure target mRNA degradation prior to gene induction by an additional auxin treatment (2 μM NAA for 4 h). Protoplast transformation and culture Protoplast transformation has been described previously [59] and was performed with minor modifications [47] . In detail, protoplasts were prepared from 3-weeks-old Arabidopsis WT plants by ventrally cutting leaves and placing them over night into enzyme solution (1.25% (w/v) Cellulase R-10, 0.3% Macerozyme R-10, 0.4 M mannitol, 20 mM KCl, 10 mM CaCl 2 , 20 mM MES (pH 5.7)). The ensuing day protoplasts were washed twice using the isotonic washing buffer W5 (2 mM MES (pH 5.7), 154 mM NaCl, 125 mM CaCl 2 , 5 mM KCl) before resuspending them in transformation buffer MMG (4 mM MES (pH 5.7), 0.4 M mannitol, 15 mM MgCl 2 ) to a final concentration of 1 × 10 5 protoplasts per ml. For standard transformations up to 40 μg of total plasmid DNAs were placed into a 2 ml Eppendorf tube and were gently resuspended with 200 μl of protoplast solution. Subsequently 220 μl of PEG solution (40% (w/v) PEG4000 in ddH 2 O containing 0.2 M mannitol and 100 mM CaCl 2 ) were added and solutions were again gently resuspended by inverting the tubes several times. After 20 min of incubation, 800 μl of washing buffer was added and protoplasts were collected by centrifugation (1 min at 300 g ). The supernatant was discarded and the protoplast pellet was taken up in 300 μl incubation buffer WI (4 mM MES (pH 5.7), 0.5 M mannitol, 20 mM KCl). For auxin treatment, protoplasts were incubated over night in WI buffer supplemented with 0.25 μM NAA (Sigma-Aldrich Chemie, Munich, Germany). In standard transactivation experiments, 9 μg of reporter plasmid, 3 μg of a NAN normalization plasmid [60] and 14 μg of an effector plasmid have been used. Concerning protoplast two hybrid analyses, 9 μg of the ProGal 4 -UAS:GUS reporter construct (B. Weisshaar, University of Bielefeld, Germany), 3 μg of the NAN normalization plasmid and 14 μg of Gal4-binding domain (BD) and/or Gal4-AD effector fusion constructs were applied. Presented data are given as relative GUS/NAN expression levels and were obtained from three biological replications and two technical replicates each. In HAT and HDAC inhibitor studies, protoplasts were cultivated for 4 h in isotonic WI buffer supplemented with or without 0.8 μM TSA (Cell Signaling Technology, USA), or 0.25 mM γ-butyrolactone (ALX-270-411; Axxora, Lörrach, Germany), prior to an additional 2 h incubation period with the inhibitors and 2 μM NAA or an adequate mock additive (DMSO). Molecular biological techniques DNA sequence analyses were performed using an ABI310 sequencer (Applied Biosystems, Darmstadt, Germany) with an ABI PRISM BigDye terminator cycle sequencing reaction kit (Applied Biosystems, Darmstadt, Germany). Vector DNA was gel extracted and prepared using commercial kits (Macherey-Nagel KG, Düren, Germany). Western analysis was performed making use of a primary polyclonal α-HA antibody from rabbit (1:700 dilution) (cat. no. sc-805, Santa Cruz, Santa Cruz, CA, USA) or a monoclonal α-MYC antibody from mouse (1:1,000 dilution) (cat. no. 2276, Cell Signaling Technology, USA) and a secondary anti-rabbit (1:10,000 dilution) (cat. no. NA934) or anti-mouse (1:7,500 dilution) (cat. no. RPN4201) immunoglobulin G conjugated with a horseradish peroxidase (GE Healthcare, Freiburg, Germany). Protein loading was quantified by Ponceau S staining or by determining ACTIN11 (At3g12110) abundance using an α-ACTIN11 antibody from mouse (1:1,000 dilution) (cat. no. AS10702, Agrisera, Sweden). Where portions of blots have been presented in the manuscript, the full blots are shown in the Supplementary Information ( Supplementary Fig. 7 ) QRT–PCR has been performed with SYBR green as described previously [55] . Data were obtained from three replicates of at least two individual plant pools and are normalized to UBQ5 (At3g62250) transcript abundance. All qRT–PCR oligonucleotide primers used are summarized in Supplementary Table 1 . Vector construction Standard DNA cloning techniques have been described previously [61] . The Pro GH3.3 :GUS reporter construct used in the transient protoplast transactivation assays was created by amplifying the promoter sequence including the 5′UTR from GH3.3 (~\n1,700 bp) from Arabidopsis WT genomic DNA by PCR using the primers listed in Supplementary Table 1 . Making use of the attached flanking restriction sites of the resulting PCR products ( Xba I, Nco I), the promoter fragment was inserted into the reporter plasmid pBT10-GUS (B. Weisshaar, University of Bielefeld, Germany). The Pro GH3.3 −300–1,700 derivative was generated accordingly using Xba I/ Nco I restriction sites. The Pro GH3.3 −300 :GUS construct was created by removing the upstream promoter region (300–1,700 bp) from the pBT10-Pro GH3.3 :GUS construct by digestion with Bsi WI and Xba I, subsequent fill-in of the resulting sticky ends with Klenow fragment (Fermentas, Germany) and blunt-end ligation of the vector. For site-directed mutagenesis of the AuxRE and GRE cis -elements within the GH3.3 promoter, the Quick Change site-directed mutagenesis kit (Stratagene, Amsterdam, Netherlands) was used following the manufacturer’s manual. The primers were designed according to: http://www.stratagene.com/qcprimerdesign and are listed in Supplementary Table 1 . The bZIP group S1 and C bZIP effector plasmids (HA, BD and AD fusions) used in the transactivation assays were described previously [47] . The entry clone for IAA3 was obtained from the REGIA TF collection [62] and for ADA2a/b from Steven J. Triezenberg, Michigan State University, USA. N-terminal truncated bZIP11 and bZIP44 constructs were created by amplifying the corresponding gene fragment from the bZIP11 and bZIP44 full-length entry clones using gateway compatible primers ( Supplementary Table 1 ). Using the Gateway technology (Invitrogen, Darmstadt, Germany), the genes stored in entry clones were transferred into the transient pHBTL-HA/AD/BD expression vectors [47] . For Co-IP experiments, the transient pHBTL-MYC expression vector was constructed. Therefore, the Pro35S:HA-gateway cassette fragment from the pHBTL-HA vector was exchanged by the Pro35S:4xMYC-gateway cassette from the binary pGWB18 vector [63] using Afl II and Hin dIII restriction enzymes. The XVE system was applied for Est-inducible expression. The gateway compatible binary pMDC7 vector [46] was used for inducible expression of amiRNA constructs. Target specific and efficient amiRNA sequences were identified using the online amiRNA design tool WMD2 ( http://wmd2.weigelworld.org ). To generate inducible overexpressors and to monitor target gene expression, a HA-tag was incorporated into the pMCD7 vector. The HA-tag was PCR amplified from the pE-HA vector [64] attaching Xho I restriction sites and inserted between the inducible promoter and the gateway attachment site of the pMDC7 vector. Chromatin immunoprecipitation ChIP was described previously [65] and was performed with minor modifications. In detail, 8 g of leaf material was incubated with cross-linking buffer (50 mM KH 2 PO 4 /K 2 HPO 4 buffer (pH 5.8), 1% (v/v) formaldehyde) for 30 min under vacuum. Cross-linking was stopped by incubating the samples in glycine buffer (50 mM KH 2 PO 4 /K 2 HPO 4 buffer (pH 5.8), 0.3 M glycine) for 15 min under vacuum followed by further washing with ice-cold water. Samples were frozen in liquid nitrogen and subsequently grinded. Nuclei extraction was performed in a cooling chamber at 4 °C. Therefore, plant material was resuspended in 24 ml ice-cold extraction buffer (1 M hexylenglycol, 50 mM PIPES-KOH (pH 7.2), 10 mM MgCl 2 , 5 mM ß-mercaptoethanol, one tablet per 10 ml complete protease inhibitor cocktail tablets, Roche) and was cleared by filtrating it through two layers of miracloth. A quantity of 1 ml of 25% Triton X-100 was added dropwise to the extract. After incubation for 15 min, nuclei were isolated by density-gradient centrifugation using a 35% percoll cushion. The nuclei pellet was resuspended in sonication buffer (10 mM Tris–HCl (pH 7.4), 1 mM EDTA (pH 8.0), 0.25% SDS and protease inhibitor) prior to sonification for 20 × 20 s. Chromatin was cleared by centrifugation for 15 min at 11,000 g , 4 °C and frozen in aliquots. For each IP, 15 μg chromatin and 2–5 μg ChIP grade antibody (Abcam, Cambridge, UK); ChIP grade α-HA (ab9110), ChIP grade Histone H3 acetyl K27 (ab4729), ChIP grade RNA polymerase II CTD repeat YSPTSPS (phosphor S5) (ab5131) or 20 μl of a GCN5-specific antiserum [18] were used. Seventy microlitres of protein A-coated magnetic beads (Invitrogen, Karlsruhe, Germany) dissolved in ice-cold extraction buffer, supplemented with protease inhibitor (Roche, Mannheim, Germany) were applied to each sample. Antibody–antigen binding was achieved during a 2 h incubation step at 4 °C and slow rotation on an Intelli-Mixer. To remove unspecifically bound proteins, beads were washed four times with washing buffer supplemented with protease inhibitor, before precipitated protein–DNA complexes were dissolved in elution buffer. Precipitated DNA was quantified by qRT–PCR using the oligonucleotide primers summarized in Supplementary Table S1 . Data were normalized to DNA input, which was quantified by ACTIN8 (At1g49240) transcript abundance. Results were obtained from two independent plant pools per line and treatment, from which 2–3 independent ChIP experiments for each antibody were performed. Co-IP assays Protocol for Co-IP assays was previously described [66] and was performed with minor modifications. In detail, 2 ml protoplasts (2 × 10 5 ml −1 ) were transfected as described in the protoplast transformation section applying 200 μg of Pro35S:HA-AtbZIP and/or Pro35S:MYC-AtADA2b effector constructs. Proteins from transfected protoplasts were extracted in a cooling chamber at 4 °C adding 0.5 ml extraction buffer (10 mM HEPES (pH 7.5), 100 mM NaCl, 1 mM EDTA, 10% glycerol, 0.5% Triton X-100 and a protease inhibitor cocktail from Roche). After lysing the cells by vigorously vortexing for 30 s, cell debris was removed by centrifugation at 11,000 g for 15 min at 4 °C. The supernatant was incubated with 2 μg of a CHIP grade α-HA antibody (ab9110; Abcam, Cambridge, UK) for 1 h at 4 °C with gentle shaking, prior to an additional incubation for 2 h with 70 μl of a prewashed, protein A-coated Dynabead/extraction buffer solution. Subsequently beads were collected using an appropriate magnet and washed four times with washing buffer (10 mM HEPES (pH 7.5), 100 mM NaCl, 1 mM EDTA, 10% glycerol, 0.1% Triton X-100 and a protease inhibitor cocktail). Bound proteins were eluted with a 5 × SDS/urea sample buffer and subjected to SDS–PAGE. Co-immunoprecipitated proteins were analysed by immunodetection using an α-HA or α-MYC antibody. The protein bands of expected molecular weights are presented. Shown are the data from one out of three Co-IP experiments, which showed comparable results. Statistics and alignments Figures and statistical tests were done applying the OriginPro 8.1 G and Statgraphics Centurion XVI software. Significant differences between multiple constructs and treatments were determined using the one-way analysis of variance test followed by a Fisher post hoc test ( P≤ 0.05) and are visualized by different letters. Significant differences between only two data sets are defined making use of the Students t -test and are labelled with asterisks (* P≤ 0.05; ** P≤ 0.01; *** P≤ 0.001). Protein sequence alignments were performed with Vector NTI 10 software (Invitrogen, Darmstadt, Germany). How to cite this article : Weiste, C. & Dröge-Laser, W. The Arabidopsis transcription factor bZIP11 activates auxin-mediated transcription by recruiting the histone acetylation machinery. Nat. Commun. 5:3883 doi: 10.1038/ncomms4883 (2014).